Development of a universal stress sensor for graphene and carbon fibres Carbon fibres are a significant volume fraction of modern structural airframes. Embedded into polymer matrices, they provide significant strength and stiffness gains by unit weight compared with competing structural materials. Here we use the Raman G peak to assess the response of carbon fibres to the application of strain, with reference to the response of graphene itself. Our data highlight the predominance of the in-plane graphene properties in all graphitic structures examined. A universal master plot relating the G peak strain sensitivity to tensile modulus of all types of carbon fibres, as well as graphene, is presented. We derive a universal value of—average—phonon shift rate with axial stress of around −5 ω 0 −1 (cm −1 MPa −1 ), where ω 0 is the G peak position at zero stress for both graphene and carbon fibre with annular morphology. The use of this for stress measurements in a variety of applications is discussed. Graphene is a one-atom-thick planar sheet of sp 2 -bonded carbon atoms stacked in a two-dimensional honeycomb lattice, and is the basic building block for carbon allotropes of any dimensionality, such as graphite, nanotubes and fullerenes [1] . It can also be considered as an infinitely large aromatic molecule [2] . Graphitic materials, including carbon fibres (CF) or multiwall nanotubes (MWNTs), are also governed in terms of their physicomechanical properties, by the anisotropy between the strong intramolecular covalent forces and the weak intermolecular (van der Waals) forces. In CF, the basic structural units (BSUs) are thought to be graphite crystals, with a lateral extension L a ∼ 2–6 nm and a stacking height L c ∼ 1–10 nm depending on the final graphitization temperature [3] , [4] . However, this view has been challenged [5] on the basis of the fact that the interplanar distance differs considerably from graphite [6] as has also been confirmed recently by high-brilliance synchrotron X-ray measurements [5] . Single-wall nanotubes (SWNT) can also be thought of as folded graphene, whereas the MWNT morphology has both graphene tubular (longitudinal direction) and graphitic (through thickness direction) characteristics. Therefore, the detailed knowledge of the mechanical behaviour of the basic graphene structural unit should yield important information on the properties not only of graphitic structures, such as graphite itself and CFs, but also of tubular structures, at least in the longitudinal direction. The entire fuselage of some modern civil aircrafts is constructed from CF composites and, in particular, polyacrylonitrile (PAN)-based CF reinforced plastic. The PAN fibre precursor, produced after wet or dry spinning of the bulk polymer [7] , has a high degree of molecular orientation and gives greater CF yield [8] . For this type of fibres, the prevalent notion is that the mechanical properties are governed by the structure and properties of the BSU [3] . However, there is no agreement as to what exactly the BSU consists of. Structures comprising elongated ribbons [9] , or crumpled and folded sheets [6] have been proposed. Another route to CF production starts from petroleum or coal tar pitch [3] , which is thermally treated above 350 °C to convert it to the well-known mesophase pitch (MPP) [3] . With reference to the development of spectroscopic stress sensors, a substantial amount of research focussed on the stress-induced alterations in the Raman spectra of a range of materials, both organic and inorganic [10] , [11] , [12] . In graphitic materials, such as CF, the variation in phonon frequency per unit of strain can provide information on the efficiency of stress transfer to individual bonds [13] . When macroscopic stress is applied to a polycrystalline CF, the resulting deformation emanates not only from bond stretching or contraction, but also from other mechanisms, such as crystallite rotation and slippage, which do not change the phonon frequency. Indeed, the higher the CF crystalline order (hence the modulus [3] ), the higher is the bond deformation, and hence, the higher is the Raman shift per unit strain [13] . The Raman G peak corresponds to the in-plane, doubly degenerate E 2 g phonon at the graphene Brillouin zone centre [14] , [15] , [16] and is present in all carbonaceous materials [17] . It is thus the ideal phonon to monitor the in-plane properties of complex graphitic structures, such as CF (see Methods for more details on Raman scattering). Previous Raman work on CFs revealed that the G peak shifts linearly with macroscopic applied uniaxial stress for various CF families of quite diverse elastic moduli [13] . Indeed, it was reported that the rate of change of G peak position with applied strain, ∂ ω /∂ ɛ , is linearly related to the CF modulus, E : ∂ ω /∂ ɛ ∝ E [13] , [18] . Given that, by definition, E is the proportionality constant between axial stress σ and strain ɛ , it follows that ∂ ω /∂ σ should take a constant value [13] , [18] for specific CF families (that is, derived from an identical precursor and processing conditions). Hence, these fibres can be considered as equal stress bodies (that is, springs in series) [19] regardless of their respective modulus. The question now is why ∂ ω /∂ σ varies when changes are brought about to the fibre precursor [18] and/or to the degree of fibre drawing within the carbonization or stabilization [13] , [18] regimes. Note that in most experiments, ∂ ω /∂ σ is estimated by performing direct ∂ ω /∂ ɛ measurements and then dividing the resulting ∂ ω /∂ ɛ by the CF tensile modulus [18] . Therefore, any underestimation of the effective optical 'skin' modulus of 13–15 nm [20] , [21] , [22] , [23] in depth will affect the results as it would effectively boost the value of ∂ ω /∂ σ [18] . However, this cannot be the only source of discrepancy as direct mechanical measurements on a PAN fibre [24] yielded a higher value of ∂ ω /∂ σ than that reported by Huang and Young [18] for fibres with approximately the same E . Axial stress applied on graphene lifts the degeneracy of the E 2 g phonon [25] , splitting the G peak into two distinct G − and G + components. The Raman intensities of the two peaks are then given by [25] : where ϕ is the angle between the strain axis and the x axis, chosen to be perpendicular to the C–C bond ( Fig. 1 ), θ in and θ out are the polarization angles of the incident and scattered light relative to the strain axis, respectively [25] , for normal incidence of light on the graphene plane. 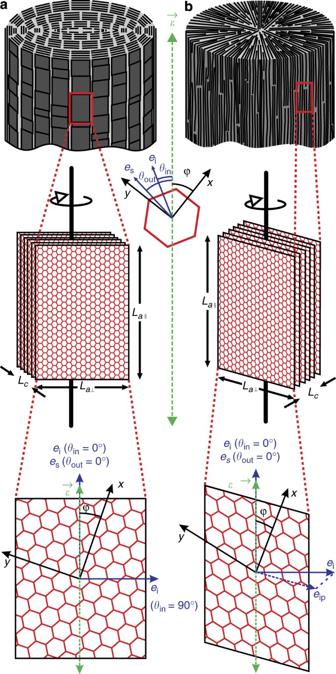Figure 1: Schematic representation of scattering geometry for onion skin and radial CFs. A simplified concept of the structure of (a) onion skin and (b) radial CFs is shown.depicts the strain axis, whereasei, andesindicate the directions of incident and scattered light, respectively.θinandθoutare the angles between the strain axis and the plane of the electric-field vector of incident and scattered light. Thexaxis is taken perpendicular to the C–C bond.ϕis the angle between the strain axis and thexaxis (that is, orientation of the graphene lattice with respect to strain).Lcis the CF crystallite thickness (that is, number of graphene layers).La||andLa⊥represent crystallite width in directions parallel and perpendicular to the fiber axis.eiis plotted in both directions, which were used in the experiments (θin=0° and 90°). In (b),eipdesignates theeivector projected onto the graphene plane, which is rotated around a vertical axis at an arbitrary angle.esis plotted only atθout=0°. Figure 1: Schematic representation of scattering geometry for onion skin and radial CFs. A simplified concept of the structure of ( a ) onion skin and ( b ) radial CFs is shown. depicts the strain axis, whereas e i , and e s indicate the directions of incident and scattered light, respectively. θ in and θ out are the angles between the strain axis and the plane of the electric-field vector of incident and scattered light. The x axis is taken perpendicular to the C–C bond. ϕ is the angle between the strain axis and the x axis (that is, orientation of the graphene lattice with respect to strain). L c is the CF crystallite thickness (that is, number of graphene layers). L a || and L a ⊥ represent crystallite width in directions parallel and perpendicular to the fiber axis. e i is plotted in both directions, which were used in the experiments ( θ in =0° and 90°). In ( b ), e ip designates the e i vector projected onto the graphene plane, which is rotated around a vertical axis at an arbitrary angle. e s is plotted only at θ out =0°. Full size image A question that needs addressing is whether the graphene orientation in CF also leads to observable phonon splitting and stress/strain-induced shifts. This is important in view of the possible use of CF as stress/strain sensors in commercial composites, in tandem to their primary role as structural reinforcements. As the average orientation of the CF-BSU with respect to the incident light is fixed during the carbonization and drawing procedures [3] , it follows that polarized Raman measurements could in principle determine the relative contribution of each G peak component. Indeed, it was long known that in CF, the full width at half maximum of the G peak (FWHM(G)) increases with tensile strain [4] , in contrast to the expectation that this should decrease following the decrease of crystallite misorientation. Hence, it is reasonable to assume that the observed broadening of the G peak in CF is an indication of phonon splitting during mechanical loading. We embarked on an experimental campaign to examine the response of the basic graphene unit present in all graphitic structures to an applied tensile stress/strain field. Two PAN-based and two pitch-derived CFs of various elastic moduli have been selected for polarized Raman measurements and the results are compared from a variety of PAN-based and pitch-based fibres reported in the literature [4] , [18] . By plotting the G peak strain sensitivity as a function of modulus for all types of CF, we have found that all data points lie within the boundaries defined by graphene itself. A universal value of—average—phonon shift rate with axial stress of around −5 ω 0 −1 (cm −1 MPa −1 ) is thus derived. Strain/stress sensitivity of the G peak of graphene Graphene monolayers were subjected to tensile loading by means of a cantilever beam (CB) apparatus. 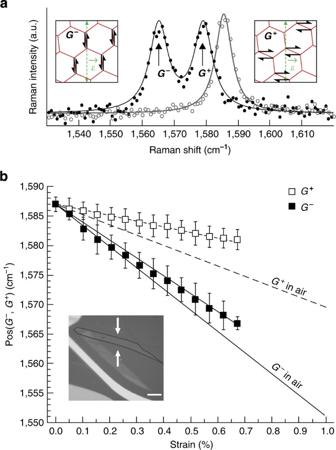Figure 2: Graphene under strain. (a) G peak Raman spectra of graphene at 0% (grey) and 1% (black) strain at 785 nm excitation. The solid curves are Lorentzian fits. The insets show the eigenvectors of theG+andG−modes25. (b)G+(empty rectangles) andG−(full rectangles) peak positions for graphene embedded in polymer beam in tension. The data points are averages from four different locations on the flake , with the error bars denoting the s.d. Labelled lines represent values calculated for suspended graphene (see text). The inset shows an optical microphotograph of the measured flake. Scale bar, 10 μm. The arrows indicate the strain orientation. Representative Raman spectra in the G peak spectral region of graphene at 0 and 1% of strain are plotted in Figure 2a and the fitted positions of the G subbands (Pos(G)) as a function of strain are shown in Figure 2b . Care was taken to measure flakes with zero residual strain to avoid non-linear effects [25] . The initial stress condition of the flake depends on fabrication (mechanical cleavage) and/or on surrounding film shrinkage due to curing. The straight lines are least-squares-fits of four sets of measurements, giving an average ∂ ω G + /∂ ɛ =−9.7×10 2 cm −1 and ∂ ω G - / ∂ ε =−31.5×10 2 cm −1 in good agreement with previous measurements employing a different loading device [25] . To derive the phonon shifts with respect to axial strain for unsupported graphene, and therefore eliminate any effect from the substrate Poisson's ratio, we first estimate the Gruneisen and the shear deformation potential parameters for the supported case, then revert to free-standing graphene [25] . Such procedure yields ∂ ω G + / ∂ ε =−17.5×10 2 cm −1 and ∂ ω G − /∂ ɛ =−36.0×10 2 cm −1 , which is comparable to −18.6×10 2 cm −1 and −36.4×10 2 cm −1 , respectively, obtained earlier [25] . Figure 2: Graphene under strain. ( a ) G peak Raman spectra of graphene at 0% (grey) and 1% (black) strain at 785 nm excitation. The solid curves are Lorentzian fits. The insets show the eigenvectors of the G + and G − modes [25] . ( b ) G + (empty rectangles) and G − (full rectangles) peak positions for graphene embedded in polymer beam in tension. The data points are averages from four different locations on the flake , with the error bars denoting the s.d. Labelled lines represent values calculated for suspended graphene (see text). The inset shows an optical microphotograph of the measured flake. Scale bar, 10 μm. The arrows indicate the strain orientation. Full size image The secular equation for the E 2 g mode of graphene under strain is [25] , [26] , [27] , [28] : where λ=( ω 2 − ω 2 0 )≈2 ω 0 Δ ω is the difference between the squared strain-dependent frequency, ω , and the squared frequency in the absence of strain, ω 0 . Solving equation (2) analytically, and ignoring terms higher than ɛ 2 , the G − and G + shifts in uniaxially strained graphene in the x direction ( ɛ xx = ɛ , ɛ yy =−ν ɛ , ɛ xy =0) are: or Inserting the estimated values of ∂ ω G + /∂ ɛ and ∂ ω G − /∂ ɛ for free graphene in equations (5) and (6), we get A =−1.23×10 7 cm −2 and B =−7.16×10 6 cm −2 in agreement with previously obtained values [25] , [28] . We now consider the stress sensitivity. For uniaxial stress, the resulting strains are given by ɛ xx = ɛ = S 11 σ and ɛ yy =−ν ɛ = S 12 σ or equivalently: where S 11 and S 12 are the compliances. Following the analysis mentioned earlier, we obtain: To derive the G peak stress sensitivity, we need the graphene compliance constants, C ij . When and (refs 29 , 30 ), inserting these S11, S12 in equations (9) and (10), we obtain ∂ ω G + /∂ σ =−1.6 cm −1 GPa −1 and ∂ ω G - / ∂ σ =−3.5 cm −1 GPa −1 . The corresponding values from experiments on an embedded flake using the CB apparatus [31] , [32] are approximately −1.7 and −3.6 cm −1 GPa −1 , whereas those derived earlier on a bare flake using the four-point-bending test [25] were −1.9 and −3.6 cm −1 GPa −1 . The agreement between the above analysis and both experimental tests is excellent and does not depend on the type of polymer beams (CB or four-point-bending) employed to load the monolayer. Strain/stress sensitivity of the G peak of CFs When a polycrystalline (turbostratic) CF is subjected to uniaxial tension, both G − and G + should be seen. Only for specific combinations of incident polarization/analysis directions, one of the two components can be suppressed [25] . In almost all CF literature (see, for example, refs 4 , 5 , 18 ), the incident polarization is along the fibre ( θ in =0°) no analyser is used and no G peak splitting is seen, but an increase in FWHM(G). We take this FWHM(G) increase as a signature of phonon splitting. To test this hypothesis, we subject our fibres to tension and examine the peak evolution with strain for θ in =0° or 90° and θ out =0°. 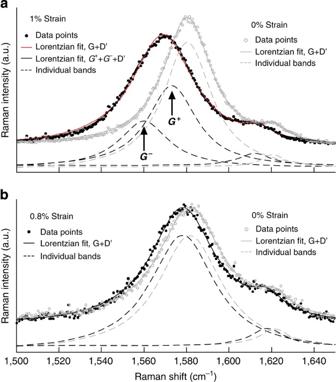Figure 3: CFs under strain. Raman G band region of (a) HM fibre at 0 (G+D', grey) and 1% (G++G−+D', black) strain and (b) of P55 fibre at 0 (G+D', grey) and 0.8% (G+D', black) strain. The lines are Lorentzian fits to the experimental spectra, in which the dashed lines stand for individual bands. The red solid line inarepresents a Lorentzian fit to the HM fibre at 1% strain using only a single G peak. For the high modulus (HM)-PAN-CF, the G peak is plotted in Figure 3a at 0 and 1% strain. For strains higher than 0.5–0.6%, the G peak can be fit with two Lorentzians (black line) better than a single Lorentzian (red line, Fig. 3a ). The two components correspond to G − and G + ( Fig. 2a ). For a tensile strain of 1% and θ in = θ out =0°, we get I ( G − )/ I ( G + ) ∼ 0.6 from a number of fibres tested ( Fig. 3a ). From equation (1) and θ in = θ out =0°, we expect I ( G − )/ I ( G + ) ∝ tan 2 (3 ϕ ), implying an average φ ∼ 13° ( Fig. 1 ). However, this result should be treated with caution even for 'onion' skin fibres, due to the presence of a disorder that can affect the measured intensities. In contrast, for the P55-CF, there is no sign of splitting at strains just before fracture ( ∼ 0.8%) indicating, as argued below, the absence of the G − component in MPP-CFs. Figure 3: CFs under strain. Raman G band region of ( a ) HM fibre at 0 (G+D', grey) and 1% ( G + + G − +D', black) strain and ( b ) of P55 fibre at 0 (G+D', grey) and 0.8% (G+D', black) strain. The lines are Lorentzian fits to the experimental spectra, in which the dashed lines stand for individual bands. The red solid line in a represents a Lorentzian fit to the HM fibre at 1% strain using only a single G peak. 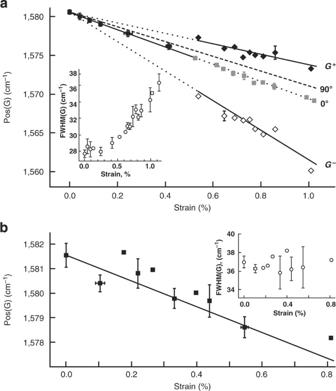Figure 4: Position of G band under strain in CFs. The position of the Raman G band of (a) HM and (b) P55-CFs. The squares represent Pos(G) fitted as a single Lorentzian forθin=0° andθout=0°. Ina, the diamonds correspond to theG+(full) andG−(empty) positions forθin=0°. The straight lines represent the least-squares fits to the experimental data (solid lines forθin=0° and dashed line forθin=90°—in the latter case the data points are not shown for the sake of clarity). The insets show the FWHM of the respective G peaks when fitted as a single Lorentzian. The error bars represent the s.d. from all measurements on the given strain level. Full size image Pos(G) as a function of strain for both the HM- and P55-CFs is plotted in Figure 4 . For the HM-CF (annular morphology), FWHM(G) increases significantly for strains higher than 0.4%, whereas the P55-CF shows no increase up to fracture. Also plotted in Figure 4 is Pos(G) for both θ in =0° and θ in =90°, with θ out =0°. For all CFs, and strains up to 0.4%, we get ∂ ω G =−11.2×10 2 cm −1 for θ in =0°, similar to what was reported earlier for similar fibres [4] , [18] , and −9.5×10 2 cm −1 for θ in =90°. However, at higher strains, by fitting two Lorentzians, we get ∂ ω G − /∂ ɛ and ∂ ω G + /∂ ɛ −18.8×10 2 cm −1 and −6.7×10 2 cm −1 ( Fig. 4a ). In contrast, the P55-CF ( Fig. 4b ), with radial morphology [18] , shows no appreciable FWHM(G) increase, hence no peak splitting. It is interesting to note that the average ∂ ω G /∂ ɛ for the P55-CF is close to that of the G + peak in the HM-CF of similar modulus. Translating this finding to the graphene plane (see Fig. 5 in ref. 25 ), prevalence of G + would imply that φ is close to zero, that is, the C–C bond is perpendicular to the fibre axis, the so-called zig-zag configuration. Figure 4: Position of G band under strain in CFs. The position of the Raman G band of ( a ) HM and ( b ) P55-CFs. The squares represent Pos(G) fitted as a single Lorentzian for θ in =0° and θ out =0°. In a , the diamonds correspond to the G + (full) and G − (empty) positions for θ in =0°. The straight lines represent the least-squares fits to the experimental data (solid lines for θ in =0° and dashed line for θ in =90°—in the latter case the data points are not shown for the sake of clarity). The insets show the FWHM of the respective G peaks when fitted as a single Lorentzian. The error bars represent the s.d. from all measurements on the given strain level. 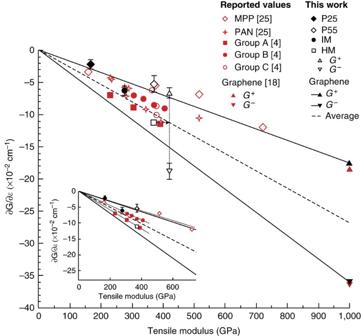Figure 5: Master plot of ∂ωG/∂ɛas a function of tensile modulus. The black solid and dashed lines correspond to fits to experimental data for graphene. The black and red triangles correspond to graphene G subbands values measured in this work and in ref.25, respectively. In red, the solid square points correspond to group A fibres, the solid circles correspond to group B, the open circles to group C4, whereas the diamonds to MPP-CFs and the stars to various PAN-CFs18. In black, data points for HM (empty square), IM (full circle), P25 (full diamond) and P55 (empty diamond) CFs measured in this work. The black empty triangles show the HM-CF G band splitting and its projection onto the graphene average line. The inset shows the ∂ωG/∂σleast-squares line fits for group A (∂ωG/∂σ=3 cm−1GPa−1), B (2.3 cm−1GPa−1) and MPP-CFs (1.5 cm−1GPa−1) as dotted lines. The other symbols in the inset have the same meaning as in the main plot. The error bars represent the s.d. from all measurements on the given fibre. Full size image Figure 5: Master plot of ∂ ω G /∂ ɛ as a function of tensile modulus. The black solid and dashed lines correspond to fits to experimental data for graphene. The black and red triangles correspond to graphene G subbands values measured in this work and in ref. 25 , respectively. In red, the solid square points correspond to group A fibres, the solid circles correspond to group B, the open circles to group C [4] , whereas the diamonds to MPP-CFs and the stars to various PAN-CFs [18] . In black, data points for HM (empty square), IM (full circle), P25 (full diamond) and P55 (empty diamond) CFs measured in this work. The black empty triangles show the HM-CF G band splitting and its projection onto the graphene average line. The inset shows the ∂ ω G /∂ σ least-squares line fits for group A (∂ ω G /∂ σ =3 cm −1 GPa −1 ), B (2.3 cm −1 GPa −1 ) and MPP-CFs (1.5 cm −1 GPa −1 ) as dotted lines. The other symbols in the inset have the same meaning as in the main plot. The error bars represent the s.d. from all measurements on the given fibre. Full size image The expected shift per unit of normal stress in fibres can be derived as follows. If both components contribute equally to the measured Raman shift, using equations (9) and (10) we get: By returning to the treatment presented in the previous section for graphene, we can estimate the theoretical value of the expression in brackets as −5 ω 0 −1 (cm −1 MPa −1 ). This is valid at least for annular morphology CFs (that is, most PAN-based CFs) and confirms the applicability of the fibre as stress sensors in a number of applications. As shown below, it also defines the mean value of phonon shift over a wide modulus range. To visualize the structural relation between graphene and CFs, a universal master plot is constructed. In Figure 5 , the ∂ ω G /∂ ɛ for graphene, the PAN-based, HM and intermediate modulus (IM) fibres, as well as the MPP-based, P55 and P25 fibres, are plotted against their nominal—bulk—tensile Young's modulus. All these data were obtained for θ in =0° and θ out =0°. Furthermore, we include data from PAN-based and MPP-CFs measured over the past 20 years [4] , [18] (see Methods for details). All CF data are contained within two boundary lines defined by the graphene G + and G − slopes −1.7 and −3.6 cm −1 GPa −1 . We also note that the data points from fibres exhibiting annular structure (classical processing route [3] ) lie below the bisector (average) line ∂ ω G /∂ σ =−2.7 cm −1 GPa −1 , also confirmed by direct stress measurements [24] . On the contrary, PAN-CFs produced by the imposition of a higher drawing ratio at the carbonization stage and at lower ultimate firing temperature (UFT) have much smaller ∂ ω G /∂ σ . A further validation of this phenomenon is given for the so-called group C fibres [4] of approximately the same modulus but of varying draw ratio [4] . In this case, the higher the extent of pregraphitization drawing, thus the lower the UFT, the smaller the ∂ ω G /∂ σ . It appears therefore that, as the CF morphology is altered by drawing from the annular ('onion') to a highly folded structure [4] , the data shift towards the G + boundary (see Fig. 5 ). The PAN-CFs from ref. 18 consist of various fibres obtained from different producers and derived through different processing conditions. Yet, their data points lie within the boundaries of the G + and G − lines as the PAN fibres mentioned above. Finally, the data for MPP-CFs with radial morphology, measured in this study and those extracted from the literature [18] , tend to conform to the G + line of slope ∂ ω G /∂ σ =−1.6 cm −1 GPa −1 . These effects can be explained by the results of the previous sections with reference to the angle φ between strain axis and C–C bond ( Fig. 1 ). As the graphene stacks in CF rotate and φ decreases towards 0° (radial morphology, Fig. 1 ), the G + peak prevails, as for equation (1) with θ in = θ out =0°. Finally, the G − and G + peaks' strain shifts of −18.8×10 −2 and −6.7×10 −2 cm −1 of the HM-CF ( Fig. 4a ), respectively, can be projected onto the average line of Figure 5 to get an estimate of the true tensile modulus of the CF optical (sampling) area. This indicates a skin modulus of some 100 GPa higher than the CF bulk modulus, in broad agreement with the previous results [18] , obtained by X-ray measurements for CF of similar morphology. Note that in the case of SWNTs, the overall phonon shift will also depend on chirality. In nanotubes, pure curvature splits the graphene E 2 g mode into two components, one parallel and one perpendicular to the tube axis [33] . Thus, by curvature only, semiconducting nanotubes will have a low frequency transverse optical G − peak and a higher frequency longitudinal optical G + peak. However, in metallic SWNTs, a further significant longitudinal optical softening takes place because of the enhanced Kohn anomaly due to electron confinement, resulting in the opposite assignment of G − and G + [33] . For relatively large diameter SWNT and MWNT (>4 nm), we could use an approach similar to that outlined above for CFs, as for very large diameters the behaviour becomes similar to that of graphene [33] , [34] . For small diameters, in particular for metallic tubes, the splitting is governed mainly by electron confinement and other effects [33] . To date, a few experiments have been reported on strained individual SWNTs with diameters ranging from 0.8 to 1.7 nm [35] , [36] , [37] . Even though, as expected, the G + and G − shift rates are generally different from graphene, there appears to be an increase of shift per stress with increasing diameter [37] up to −2.6 cm −1 GPa −1 (refs 35 , 37 ), in agreement with the average trend in Figure 5 . In summary, the knowledge of the G peak shift and splitting with uniaxial strain in graphene was used to interpret the mechanical response of various CF types. For polarized measurements, accurate determination of the G peak shift and splitting with stress is a route to evaluate the average orientation of the graphene units (or stacks) with respect to the fibre (strain) axis and, in certain cases, to the optical skin modulus. By comparing the results derived for graphene and CFs, a universal plot was constructed relating the G peak shift to stress or strain for all graphitic materials. In other words, the phonon deformation (atomic scale) scales to the imposed stress (macroscale) in an identical manner for a range of CFs with different moduli but related morphologies. We estimate a universal value of average G peak shift with stress approximately −5 ω 0 −1 cm −1 MPa −1 regardless of modulus. This could lead to sensors within structures (airframes and so on) made of CF composites, converting Raman shifts into stress. In the aerospace field, this in-flight monitoring would be more preferable and complementary to the current postflight inspections ( http://www.asnt.org ). CFs The HM fibre has 7 μm diameter and 370 GPa bulk modulus. This is produced by conventional manufacturing technologies [3] , [4] . Acrylic filaments were wet-spun and drawn in hot water and saturated steam to a total draw ratio of 14, to yield a final diameter of ∼ 12 μm. The filaments were stabilized in hot air to a density of ∼ 1.38−1.40 gcm −3 using a rising-ramped temperature regime (225–245 °C). Primary carbonization was carried out using a maximum temperature of 950 °C, whereas secondary carbonization and graphitization were at UFT=2,600 °C. No additional drawing processes were carried out. During stabilization, the filaments were held at constant length. During carbonization and graphitization, a 5% shrinkage was allowed. The IM fibre has 5-μm diameter and 270 GPa bulk modulus. Acrylic filaments were wet-spun and drawn as described above. The filaments were then subjected to a multistage prestabilization drawing at temperatures up to 270 °C, followed by stabilization as described above. Carbonization and graphitization were carried out with the filaments held at constant length at UFT=1,750 °C. Two commercial MPP fibres with E ∼ 167 GPa (P25) and 371 GPa (P55) sourced from Cytec Industries were also tested. These use MPP derived from petroleum or coal tar [3] . The production of pitch-based CFs involves melt spinning of pitch precursor fibres, stabilization (oxidation), carbonization and graphitization [3] . Group A and group B fibres in Figure 5 were also manufactured with the processes mentioned above for HM and IM fibres. Group C consists of three 6-μm-diameter fibres of similar Young's modulus, but with different morphologies [4] . Acrylic filaments were also treated as in group A fibres, but different drawing procedures were used in the stabilization (up to 270 °C) and carbonization regimes (up to 950 °C). Thus, the higher the amount of fibre drawing, the lower is the UFT required to get the 370 GPa modulus [4] . As shown in Figure 5 , by altering the drawing procedure and reducing the UFT, ∂ ω G /∂ σ shifts to lower values ( G + dominance). The data from a range of MPP-CFs measured by Huang and Young [18] are also shown in Figure 5 . Graphene Graphene monolayers were prepared by mechanical cleavage from natural graphite (Nacional de Grafite) and transferred onto the poly methyl methacrylate acetate (PMMA) CB covered by a ∼ 200-nm-thick layer of SU8 photoresist (SU8 2000.5, MicroChem). A thin layer of S1805 photoresist (Shipley) was spin coated on top. The beam has a total thickness 2.9 mm and width 12.0 mm. The graphene flake was located at 12.97 mm from the beam end. The flake's dimensions are 6×56 μm 2 , with the shorter side parallel to the strain axis. Raman spectroscopy Apart from the G band mentioned in the main text, other Raman features can be traced in carbonaceous materials. The D peak is due to the breathing modes of sp 2 rings and requires a defect for its activation [16] , [38] . It comes from the transverse optical phonon branch (TO) around the K point of the Brillouin zone [16] , [38] , [39] is active by double resonance (DR) [40] and is strongly dispersive with excitation energy due to a Kohn Anomaly at K [39] . DR can also take place intravalley, that is, connecting two points belonging to the same Dirac cone around K or K ′. This gives rise to the so-called D′ peak, which appears around 1620 cm −1 in defected graphite and CFs measured with visible excitation. The 2D peak is the second order of the D peak. This is a single peak in single-layer graphene, whereas it splits into four in bilayer graphene, reflecting the evolution of the band structure [15] . The 2D′ peak is the second order of the D′ peak. Because both 2D and 2D′ originate from a process where momentum conservation is satisfied by two phonons with opposite wavevectors, q and −q , they do not require the presence of defects for their activation, and are thus always present [15] . Indeed, high-quality graphene shows the G, 2D and 2D′ peaks, but not D and D′ [15] . Unlike the G peak, the 2D band shows a significant evolution in shape with the number and orientation of the graphene layers [15] , as well as broadening [25] , [41] or splitting [41] , [42] according to the uniaxial strain orientation with respect to the graphene unit cell. However, while amorphous carbons or CFs of low modulus show a broad and almost featureless 2D peak [14] , [38] , owing to the additional effect of defects in the DR process, the G peak, even though broader compared with graphene [14] , [38] , is always present, being just due to the relative motion of carbon atoms and not requiring the presence of sp 2 rings [14] , [38] . Hence, the G peak is ideal for comparative studies of in-plane stress and strain between different graphitic materials. MicroRaman (InVia Reflex) spectra were recorded with 785 nm (1.58 eV) excitation, with power kept below 0.85 mW to avoid heating. Such a wavelength was used to suppress the polymer coating fluorescence. A ×100 objective with numerical aperture 0.9 is used, with a ∼ 1×2 μm 2 spot size. The polarization of the incident light was kept parallel to the applied strain. The spectra were first baseline subtracted, then the spectrum of bare substrate was subtracted. All bands were fitted with Lorentzians. FWHM(G) for the unstressed graphene is ∼ 6–8 cm −1 . CF MicroRaman spectra were measured at 514.5 nm (2.41 eV) with a laser power below 1.1 mW. A ×80 objective with numerical aperture 0.75 is used, and the spot size is estimated ∼ 1 μm 2 . The data are collected in back scattering with a triple monochromator and a Peltier-cooled charge-coupled device detector. The incident polarization was either parallel ( θ in =0°) or perpendicular ( θ in =90°) to the applied strain axis. The scattered polarization was selected to θ out =0°. Individual CF in air were bonded to the jaws of a small straining rig, with their axes aligned parallel to the stretching direction to ±5°. The gauge lengths of the fibres were fixed to 25 mm and the fibre extension measured to ±1 μm. The spectra were taken close to the middle of the fibre, and five measurements were averaged for each step. The HM-CF ∂ ω G /∂ ɛ shift rate was determined from eight independent experiments at θ in =0° and five with θ in =90°, using at least three measurements at every strain level. The strain was increased in steps 0.05–0.2% up to failure at 0.8–1.1%. All spectra were fitted with Lorentzians. For θ in =0°, the least-squares fits of Pos(G) versus ɛ were performed on every experiment and then averaged giving ∂ ω G /∂ ɛ of −11.2±0.7×10 2 cm −1 , as well as on all data giving ∂ ω G /∂ ɛ of −11.2±0.3×10 2 cm −1 . For θ in =90°, the least-squares fit of Pos(G) versus ɛ was performed on all acquired data giving ∂ ω G /∂ ɛ of −9.5±0.3×10 2 cm −1 . For the G peak deconvolution, six sets of experiments with longer accumulation times were performed. FWHM ( G + , G − ) were kept equal during the deconvolution, and values between 28 and 29 cm −1 were obtained consistently, corresponding to the CF FWHM(G) at zero strain. Because of statistically small differences in the coefficient of determination values ( R 2 ) between fits using one or two Lorentzians, the quality of the fits was also assessed from the evolution of the F -values from the analysis of variance test. The F -value is defined as where SS stands for sum of squares, DF for degrees of freedom, as obtained from regression (reg) and residual (res) least-squares values [43] . For a particular experiment, no significant difference in F -values was observed until a strain ∼ 0.5–0.6%. From this point onwards, the F -value for the single G peak progressively lowers in comparison with the G + , G − fit. The IM-CF ∂ ω G /∂ ɛ shift rate was obtained from two independent experiments, using three measurements at every strain level. The strain was increased in steps <0.1% up to failure at ∼ 0.9%. The spectra were fitted using Lorentzian D, G and D′ bands. The least-squares fit on all acquired data gives ∂ ω G /∂ ɛ =−6.2±0.8×10 2 cm −1 . The P25-CF ∂ ω G /∂ ɛ shift rate was obtained from two independent experiments, using three measurements at every strain level. The strain was increased in steps <0.1% up to failure at ∼ 0.75%. The spectra were fitted using Lorentzian D, G and D′ bands. The least-square fit on all acquired data gives ∂ ω G /∂ ɛ =−2.15±0.86×10 2 cm −1 . The P55-CF ∂ ω G /∂ ɛ shift rate was determined from five independent experiments, using at least three measurements at every strain level. The strain was increased in steps <0.1% up to failure at 0.55–0.8%. The spectra were fitted using Lorentzian D, G and D' bands. The least-squares fits on every experiment and averaged give ∂ ω G /∂ ɛ =−5.26±1.3×10 2 cm −1 , whereas on all data give ∂ ω G /∂ ɛ =−5.28±1.6×10 2 cm −1 . How to cite this article: Frank, O. et al . Development of a universal stress sensor for graphene and carbon fibres. Nat. Commun. 2:255 doi: 10.1038/ncomms1247 (2011).